Nanomechanical cleavage of molybdenum disulphide atomic layers The discovery of two-dimensional materials became possible due to the mechanical cleavage technique. Despite its simplicity, the as-cleaved materials demonstrated surprising macro-continuity, high crystalline quality and extraordinary mechanical and electrical properties that triggered global research interest. Here such cleavage processes and associated mechanical behaviours are investigated by a direct in situ transmission electron microscopy probing technique, using atomically thin molybdenum disulphide layers as a model material. Our technique demonstrates layer number selective cleavage, from a monolayer to double layer and up to 23 atomic layers. In situ observations combined with molecular dynamics simulations reveal unique layer-dependent bending behaviours, from spontaneous rippling (<5 atomic layers) to homogeneous curving (~ 10 layers) and finally to kinking (20 or more layers), depending on the competition of strain energy and interfacial energy. Mechanical cleavage technique, also known as the Scotch-tape method, has resulted in the discovery of two-dimensional (2D) crystals. It is a rather crude procedure, but, surprisingly, the produced samples demonstrated excellent quality and performance [1] , [2] , [3] , [4] , [5] , [6] , [7] . The simplicity of the Scotch tape method has initiated a booming research on graphene and other 2D materials. A rich family of such materials has been discovered, such as boron nitride (BN), molybdenum disulphide (MoS 2 ), niobium diselenide (NbSe 2 ) and Bi 2 Sr 2 CaCu 2 O x (ref. 7 ). However, the atomic processes of the micromechanical cleavage are still poorly understood. How will the atomically thin films behave during the cleavage and under the large bending conditions? Will they bend as a whole plate or will the interlayer sliding occur? Will they lose structural stability under severe bending deformation? These concerns call for a direct investigation into the initial stage of the mechanical cleavage process. One particularly promising application for the 2D crystals is flexible electronics, because of their strong in-plane bonding and high flexibility [8] , [9] , [10] , [11] , [12] , [13] . MoS 2 atomic layers are competitive candidates with suitable electronic structures [14] , [15] , [16] . Bulk MoS 2 is a layered semiconductor with an indirect band gap of ~1.29 eV. However, recently it has been demonstrated that MoS 2 monolayers have direct band gaps of ~1.8 eV with a strong photoluminescence [14] , [15] . In addition, the MoS 2 -based field effect transistors have shown outstanding performances with high ON/OFF ratios [6] . Moreover, high-performance MoS 2 thin-film transistors and gas sensors have been fabricated on flexible substrates [10] , [11] , [12] , [13] . It is important to study the 2D-MoS 2 mechanical properties for their reliable applications in flexible electronic devices. Bertolazzi et al . [5] reported fracture strength as high as 23 GPa at an effective strain of 11%, indicating that the 2D-MoS 2 could be almost defect free. The elastic properties were studied by Castellanos-Gomez et al . [16] who reported extraordinary high Young’s modulus E =0.33±0.07 TPa for the freely suspended 5–25 layers thick MoS 2 nanosheets. However, despite the above-mentioned notable progress, there have been no reports regarding the mechanical behaviour of the MoS 2 atomic layers under bending and folding conditions, although this ultimately determines the mechanical reliability of the flexible electronic devices made of such 2D semiconductors. In this work, we design an in situ transmission electron microscopy (TEM) probing technique [17] , [18] , [19] , [20] to investigate the initial stages of the 2D crystal cleavage, which is defined here as the ‘nanomechanical cleavage’, using MoS 2 atomic layers as a model material. By precisely manipulating an ultra-sharp metal probe to contact the pre-existing crystalline steps of the MoS 2 single crystals, atomically thin flakes are delicately peeled off, selectively ranging from a single, double to more than 20 atomic layers. The mechanical behaviours of the MoS 2 atomic layers during cleavage, bending and folding processes are investigated in situ . It is found that the mechanical behaviours are strongly dependent on the number of layers. Combination of in situ TEM and molecular dynamic (MD) simulations allows us to thoroughly investigate a transformation of bending behaviour from homogeneous curving to kinking. Growth and structure of MoS 2 atomic layers MoS 2 crystals for the in situ TEM nanomechanical cleavage experiments were grown by using a CVD method [21] . As shown in the scanning electron microscopy (SEM) image of Fig. 1a , triangular crystals were uniformly distributed on a SiO 2 /Si substrate over a large area. Most of them are made of monolayers; however, the by-products having multiple layers were chosen as the target material for our in situ experiments. A plane view of a MoS 2 crystal is demonstrated in a high-angle annular dark-field (HAADF) scanning transmission electron microscope (STEM) image ( Fig. 1b ), revealing a clean surface. Atomic steps are observed at the crystal edges, which are flat and open, rather than rolled up. A high-resolution STEM image is demonstrated in Fig. 1c , where the contrast is proportional to the square of the atomic number. Both molybdenum and sulphur atoms’ positions can individually be resolved to form hexagonal patterns with the Mo-Mo and Mo-S distances of ~3.1 Å and ~1.8 Å, respectively. 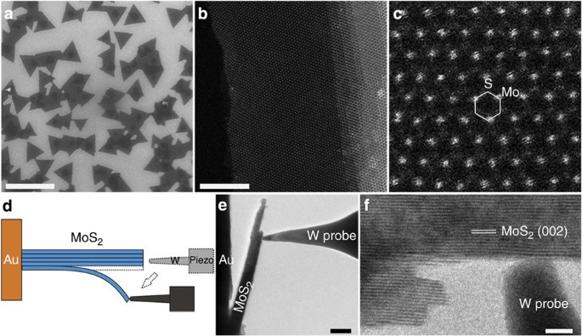Figure 1: Nanomechanical cleavage by using thein situtransmission electron microscope probing method. (a) Scanning electron microscope image of the grown molybdenum disulphide (MoS2) triangle-shaped single crystals. (b) High-angle annular dark-field image of a few-layer MoS2crystal clearly revealing the atomic steps at the edge. (c) High-resolution scanning transmission electron microscope image of the MoS2crystal. Both the Mo and S atoms could be clearly resolved. (d) Schematic of the experimental setup. An edge-on oriented MoS2crystal is placed at the stage. A tungsten tip is controlled to selectively contact, cleave and bend the MoS2atomic layers. (e) A TEM image of a tungsten nanoprobe in contact with the MoS2crystal. (f) A HRTEM image of the tungsten tip against the MoS2crystal, where the MoS2(002) atomic steps are clearly resolved. Scale bars, 5 μm,a; 5 nm,b; 50 nm,e; and 5 nm,f. Figure 1: Nanomechanical cleavage by using the in situ transmission electron microscope probing method. ( a ) Scanning electron microscope image of the grown molybdenum disulphide (MoS 2 ) triangle-shaped single crystals. ( b ) High-angle annular dark-field image of a few-layer MoS 2 crystal clearly revealing the atomic steps at the edge. ( c ) High-resolution scanning transmission electron microscope image of the MoS 2 crystal. Both the Mo and S atoms could be clearly resolved. ( d ) Schematic of the experimental setup. An edge-on oriented MoS 2 crystal is placed at the stage. A tungsten tip is controlled to selectively contact, cleave and bend the MoS 2 atomic layers. ( e ) A TEM image of a tungsten nanoprobe in contact with the MoS 2 crystal. ( f ) A HRTEM image of the tungsten tip against the MoS 2 crystal, where the MoS 2 (002) atomic steps are clearly resolved. Scale bars, 5 μm, a ; 5 nm, b ; 50 nm, e ; and 5 nm, f . Full size image Nanomechanical cleavage experimental configurations To perform the in situ TEM probing and nanomechanical cleavage experiments, the MoS 2 crystals were loaded in edge-on orientation, as shown in the schematic ( Fig. 1d ) and corresponding TEM image ( Fig. 1e ). A typical sample was about 32 nm in thickness and 380 nm in length. An ultra-sharp tungsten tip was manipulated by a piezoelectric motor to approach and contact a MoS 2 single crystal. As shown in the HRTEM image ( Fig. 1f ), there are pre-existing atomic steps at the crystal surface; therefore, the tungsten probe with a tip diameter as small as ~10 nm could be manipulated to contact the crystalline edges with a selected number of layers. By using this method, a layer-number-selective cleavage of the MoS 2 atomic layers was realized. Single-, double-, triple- and multilayers with a thickness of up to 23 atomic layers were successfully cleaved. Nanomechanical cleavage of monolayer MoS 2 The nanomechanical cleavage process of a monolayer MoS 2 is presented in Fig. 2a–d and Supplementary Movie 1 . Initially, there was a single-layer edge protruding from the MoS 2 crystal, which therefore made it possible to contact only the outermost single layer ( Fig. 2a ). After the contact, the probe was moved at an inclined angle, as marked by the black arrow, causing the single layer to attach to the probe and to be peeled off, and to bridge the nanoprobe and the ‘mother’ crystal ( Fig. 2b ). It is noted that the peeled-off MoS 2 monolayer was naturally curved, consistent with the previous theoretical and experimental works on the intrinsic rippling of 2D crystals [22] , [23] , [24] . By moving the probe away, the MoS 2 monolayer flake could be stretched and ultimately separated from the mother crystal ( Fig. 2b,c ). The insets in Fig. 2b,c demonstrate the snapshots of the corresponding MD simulations, where the profiles of simulated MoS 2 layer agree well with the HRTEM images. The simulations confirmed that the smoothly curved profile in Fig. 2b is within elastic regime. When the flake was detached, the edge was perpendicularly attached to the surface atomic step ( Fig. 2c ). HRTEM image of the MoS 2 monolayer taken before its separation is shown in Fig. 2d . MoS 2 (100) stacking order could be clearly resolved, indicating the high crystallinity. The inset of Fig. 2d demonstrates the triple-layer atomic structure, with a molybdenum atomic layer sandwiched by two sulphur atomic layers. The free-standing monolayer tends to fold up, as demonstrated using dots at the periphery lines. This also coincides with the formation of spontaneously curved edge when the monolayer was detached from the crystal ( Supplementary Movie 1 ). The spontaneous folding suggests the importance of van der Waals forces for the mechanical behaviour of 2D crystals. Interestingly enough, after initial isolation from the mother crystal, the MoS 2 monolayer could be readily restacked onto the surface of the crystal, as presented in Fig. 2e–h and Supplementary Movie 2 . First, a point contact was established between the MoS 2 monolayer and the crystal surface ( Fig. 2e ). Second, by pushing the probe, the monolayer was easily bent and formed a plane contact with the surface ( Fig. 2f ), indicating the re-establishment of crystalline stacking due to the van der Waals interactions. After that, by moving the probe parallel to the crystal surface, the MoS 2 monolayer could smoothly slip along the surface, as indicated by a change in distance between the contact point and the crystal edge that reduced from 25.5 to 8.3 nm. Finally, by pushing the probe towards the crystal, the cleaved MoS 2 monolayer was almost completely restacked onto the surface. As shown by the inset profile along the arrow in Fig. 2h , the distance between the MoS 2 monolayer and the crystal surface became ~0.65 nm, exactly the same as the interlayer distance of the initial crystal. Therefore, the nanomechanical cleavage was reversible, and no structural defects were introduced to the monolayer MoS 2 . This reversibility can explain the high quality and carrier mobility in the mechanically exfoliated 2D samples, such as graphene and MoS 2 atomically thin films [1] , [6] . 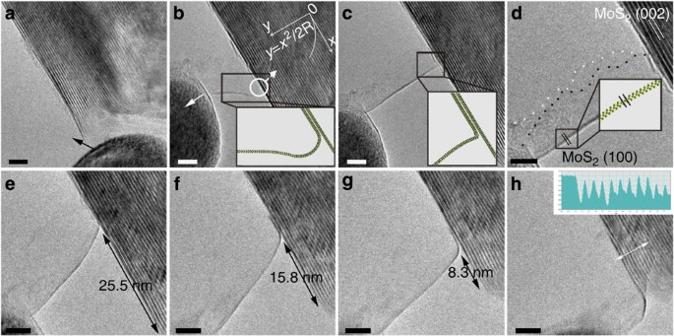Figure 2: Nanomechanical cleavage of a monolayer MoS2. (a–c) The initial contact (a), intermediate peeled-off and bent (b), and stretched (c) states of a monolayer MoS2. (d) HRTEM image of the cleaved monolayer MoS2, revealing the (100) atomic stacking order, as well as the MoS2(002) lattice fringes of the ‘mother’ crystal. The modelled atomic structures of peeled-off MoS2layer are presented in the insets ofb–d. (e–h) The movement of the cleaved monolayer MoS2on the surface of the ‘mother’ crystal, showing high reversibility during the nanomechanical cleavage. The inset inhis a profile along the arrow demonstrating the same interlayer distance of the cleaved monolayer with that of the ‘mother’ crystal. Scale bars, 5 nm, except ford(2 nm). Figure 2: Nanomechanical cleavage of a monolayer MoS 2 . ( a – c ) The initial contact ( a ), intermediate peeled-off and bent ( b ), and stretched ( c ) states of a monolayer MoS 2 . ( d ) HRTEM image of the cleaved monolayer MoS 2 , revealing the (100) atomic stacking order, as well as the MoS 2 (002) lattice fringes of the ‘mother’ crystal. The modelled atomic structures of peeled-off MoS 2 layer are presented in the insets of b – d . ( e – h ) The movement of the cleaved monolayer MoS 2 on the surface of the ‘mother’ crystal, showing high reversibility during the nanomechanical cleavage. The inset in h is a profile along the arrow demonstrating the same interlayer distance of the cleaved monolayer with that of the ‘mother’ crystal. Scale bars, 5 nm, except for d (2 nm). Full size image Nanomechanical cleavage of double and triple layers of MoS 2 By selecting the MoS 2 edges with a different number of protruding atomic layers, double and triple layers of MoS 2 were successfully cleaved from the MoS 2 crystal, as demonstrated in Supplementary Figs 1,2 and Supplementary Movies 3,4 . A double-layer MoS 2 as long as 155 nm was cleaved, as illustrated in Supplementary Fig. 1 and Supplementary Movie 3 . It was worth noting that at the beginning of the cleavage process, observations suggested six layers rather than two ( Supplementary Fig. 1a ). This is because of the mechanical contact with the probe, which led to the edge bending, rolling and crumpling. Under stretching, the crumpled MoS 2 sheet became flat, and a double layer lattice became apparent ( Supplementary Fig. 1d ). Similar process and ability to recover from severe deformations were demonstrated for a triple-layer MoS 2 ( Supplementary Fig. 2 ). The extraordinary ability to restore deformed structures demonstrates the high flexibility of the MoS 2 atomic layers, which is crucial for their applications in flexible electronics. The minimum bending radius for the inner layer of double and triple MoS 2 was about 3.0 nm and 3.1 nm, respectively. A common feature during bending was spontaneous rippling ( Supplementary Figs 1c and 2d ), which was attributed to thermal fluctuations [22] , [23] , [24] . Nanomechanical cleavage of 5- and 11-layer MoS 2 In our experiments, it was found that the mechanical behaviours of the MoS 2 atomic layers had been closely dependent on the number of layers (thickness) of the flakes. In the following section, the mechanical behaviour of comparatively thick MoS 2 stacks is discussed. The number of layers ranges from 5 to 11 in the corresponding experiments. In contrast to the relaxed ripples and folded-up configurations in the mono-, double- and triple-layer MoS 2 , such flakes were more rigid, as demonstrated by the straight profile during the bending process ( Fig. 3 , Supplementary Fig. 3 , and Supplementary Movies 5,6 ). This change is plausible, because a thicker membrane with a larger bending stiffness will have smaller displacements due to thermal fluctuations according to the relation <h 2 > ∝ TL 2 / k , where L is the size of the sample and k is the bending rigidity [25] , [26] . It is worth noting that, for the 5-layer MoS 2 , when the flake was released from the probe, it kept the bent configuration and was attached to the surface of the ‘mother crystal’, again indicating the importance of van der Waals forces for the stability and mechanical behaviours of the ultrathin crystals. 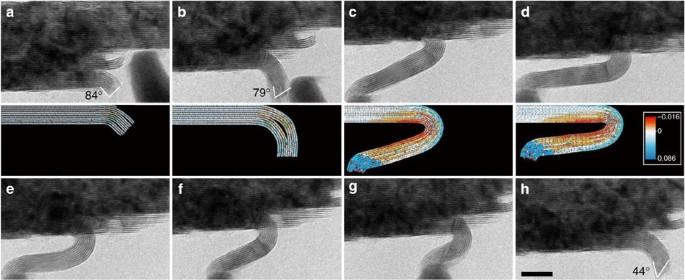Figure 3: Nanomechanical cleavage of an 11-layer MoS2. (a) Initial contact and cleavage along the MoS2(002) interlayer space. (b–d) Attaching an 11-layer MoS2to the tungsten tip and its dragging along the surface of the MoS2single crystal. The simulated structures are presented below the corresponding experimental images. The strain distribution is shown in colour: red and blue colours correspond to compressive and tensile strains, respectively. (e–h) Reverse process of the peeling process. It is reversible except the contact area with the tungsten probe. The TEM images are taken at the same magnification with the scale bar, 10 nm. Figure 3: Nanomechanical cleavage of an 11-layer MoS 2 . ( a ) Initial contact and cleavage along the MoS 2 (002) interlayer space. ( b – d ) Attaching an 11-layer MoS 2 to the tungsten tip and its dragging along the surface of the MoS 2 single crystal. The simulated structures are presented below the corresponding experimental images. The strain distribution is shown in colour: red and blue colours correspond to compressive and tensile strains, respectively. ( e – h ) Reverse process of the peeling process. It is reversible except the contact area with the tungsten probe. The TEM images are taken at the same magnification with the scale bar, 10 nm. Full size image Figure 3 and Supplementary Movie 6 present the detailed forward and reverse processes of the nanomechanical cleavage of an 11-layer MoS 2 . The original structure of the crystal is the same as that in Fig. 1f , in which the atomic steps are almost vertical to the MoS 2 (002) lattice fringes. After the initial contact and a small degree of bending, the angle became ~84° and then ~79°, indicating the interlayer sliding rather than bending as a whole plate ( Fig. 3a,b ). On further bending and cleaving, the angle between the edge and the MoS 2 (002) planes remained unchanged ( Fig. 3c–g ), indicating that the contact with the probe prohibits the interlayer sliding. In the meantime, strain contrast was observed at the transition portion between the bent and straight areas in Fig. 3c–g . Note that even with 11 atomic layers the MoS 2 sheet demonstrated high flexibility. It was bent with a radius of curvature of ~4.5 and~1.3 nm for the middle and inner layers, respectively. After release from the probe, the cleaved MoS 2 thin flake recovered to the original configuration except for the contact area. A plastic deformation was recorded close to the contact area with the angle between the edge and the MoS 2 (002) planes ~44°. Thus, the nanomechanical cleavage is largely reversible except for the contact area with the probe, and the layer damage is due to the point contact and stress concentration. MD simulations were performed for the 11-layer MoS 2 with the geometrical parameter inputs matching the experimental data ( Supplementary Movie 7 ). The edge atoms of the layers were fixed to reflect the adhesion between the tip and the sample during the cleavage process, except for the initial and final contact stages, where the MoS 2 layers became free of the probe. After that the fixed edge atoms were moved step by step, following the experimental direction. As in the previous case, a good agreement between simulated and experimental images was reached. Because of the constriction on the probe, the MoS 2 layers could not slide freely under bending, and delamination of the layers was observed, as marked in the inset of Fig. 3b , consistent with a previous theoretical work on the bending-induced delamination of van der Waals solids [27] . Under further bending, the delamination vanished due to the redistribution of the stresses in Fig. 3c,d . There were two areas with concentrated strain: one is the contact area with the probe and the other is the bent area. At the site close to the probe, all the layers are under tensile stress due to the adhesion and stretching of the probe, as indicated by the blue colour. In contrast, the site of the bent area demonstrates tensile and compressive stresses on the outer and inner surfaces, respectively. This result is consistent with the in situ observations that during the contact and cleavage process the interlayer sliding could not occur freely due to the constriction of the MoS 2 -probe interface. Therefore, while the free standing MoS 2 atomic crystals can easily slide during bending, the actual deformation process also depends on the boundary conditions. Nanomechanical cleavage and kinking of 23-layer MoS 2 We further investigated the bending process of a 23-layer MoS 2 flake ( Fig. 4 and Supplementary Movie 8 ). It was thick enough to directly measure the forces during the cleavage process; therefore, the experiments were performed using an in situ atomic force microscopy (AFM)-TEM holder. In contrast to the smoothly bent configurations for the thinner stacks, the 23-layer MoS 2 formed discrete kinks during bending, as marked by the white arrows. Accordingly, abrupt force drops were recorded, as presented in Fig. 4h . Interestingly, the kinks appeared periodically, at the bending angles of around multiples of 20°, such as 23.2°, 39.2°, 19.6° and 39.0°, as marked in Fig. 4 . It is noticed that even with the kink appearance, the whole process is largely reversible. After the separation from the AFM probe, delamination was observed only at the contact, due to the stress concentration at the contact ( Fig. 4g ). A simplified model of the MoS 2 film was adopted to simulate the process ( Supplementary Movie 9 ). At the initial state the film and the probe were brought together at a distance of chemical bond (<2.5 Å), and part of the film layers was left unbounded in accordance with the experimental conditions ( Fig. 4a ). Tangential movement of the probe led to sample cleavage. After the initial contact, the crystal transformed from the free unloaded to the compressed state, as indicated by the colour change from white to red. After that the compressed layers were elastically buckled, and the deformation was then concentrated at the buckled area. With further contact and tangential movement of the AFM probe, the layers were markedly bent and kinking took place. The geometry difference in a simulated model and experimental structure does not allow us to directly compare the calculated and in situ TEM recorded data. However, the theoretical model does capture the main experimental characteristics. The experimental force–time curve can be compared with calculated energy-simulation steps. In both plots, the observed and simulated spontaneous kink formations are represented by pronounced peaks. 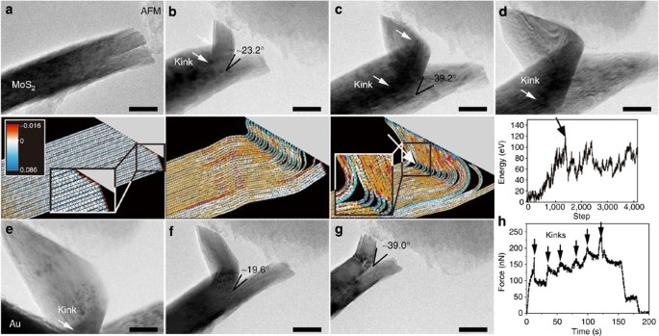Figure 4: Nanomechanical cleavage and force measurements on a 23-layer MoS2. (a–d) Forward contacting, peeling and bending of the 23-layer MoS2, with abrupt kink formation. (e–g) Reverse process of the cleavage process, leaving traces of delamination close to the contact point. (h) Force–time curve for the whole process, with abrupt force drops corresponding to the moments of kink formation. The simulated structures are presented below the corresponding experimental images. The strain distribution is shown in colour: red and blue colours correspond to compressive and tensile strains, respectively. Scale bars, 20 nm. Figure 4: Nanomechanical cleavage and force measurements on a 23-layer MoS 2 . ( a – d ) Forward contacting, peeling and bending of the 23-layer MoS 2 , with abrupt kink formation. ( e – g ) Reverse process of the cleavage process, leaving traces of delamination close to the contact point. ( h ) Force–time curve for the whole process, with abrupt force drops corresponding to the moments of kink formation. The simulated structures are presented below the corresponding experimental images. The strain distribution is shown in colour: red and blue colours correspond to compressive and tensile strains, respectively. Scale bars, 20 nm. Full size image Obviously, the bending behaviours of the MoS 2 atomic layers during cleavage are closely related to the number of layers, as summarized in Supplementary Table 1 . For the bulk layered materials such as MoS 2 , one common deformation mechanism is the formation of kinks [28] , [29] . It is noted that, for the thin 2D MoS 2 layers ( ⩽ 11 layers), they bend with the absence of kinking, even when the layers are bent to ultimately small radii (1.3~3.0 nm). The force balance of such bent MoS 2 monolayer has been analysed. The equilibrium shape is determined by the balance between the forces applied by the nanoprobe and the non-covalent dispersion forces in the vicinity of the contact—same forces that constitute the surface energy. If these van der Waals forces depend on the interlayer distance y as f(y) , then the specific surface energy γ can be written as . Near its minimum ( x = y =0 and dy / dx =0) at the contact point the bent layer shape can be described by the next quadratic term y=x 2 /2R , with R being the radius of curvature. Because of this curvature, there is a torque D(1/R) , where D =27 eV Å 2 atom −1 is the bending stiffness of MoS 2 monolayer [30] . In equilibrium, this torque must be balanced by the opposite moment produced by the distributed van der Waals forces near the contact point at x ⩾ 0, so we have D(1/R) =∫ xf ( x 2 /2 R ) dx = R ∫ f ( y ) dy = R·2 γ, and therefore, γ= D /2 R 2 . In macroscopic studies, the same relationship can be derived by energy analysis [31] , but the force approach here permits straightforward generalization for the monolayers investigation. The fitting and calculation of the curvature radius near the contact point are presented in Supplementary Fig. 4 . Moreover, the radius of curvature was calculated to be ~1.5 nm. Accordingly, the specific surface energy of MoS 2 monolayer is calculated to be ~0.06 eV atom −1 or ~0.11 N m −1 . Determination of the surface energy is fundamentally important for various processes, such as catalysis and lubrication. Previously, the specific surface energy of MoS 2 has mainly been investigated by theoretical calculations. In early publications, comparatively high values such as 0.26 and 0.28 N m −1 were reported [32] , [33] . However, the specific surface energy of MoS 2 was derived from liquid exfoliation processes [34] , [35] to be ~0.07 N m −1 . Recently, a more accurate random-phase approximation (RPA) method was adopted for the calculations of the binding energy of the van der Waals bonding in layered compounds [34] . Interlayer binding energies for a large number of layered compounds, including MoS 2 , were calculated to be around 20 meV Å −2 (~0.32 N m −1 ), with the specific surface energy being half of that value (~0.16 N m −1 ) [34] . Thus, our directly measured value is reasonably consistent with the most accurate RPA calculations currently available. For the multi-layer MoS 2 flakes, an important issue is whether the layers slide or the sample will bend as a plate. Shen et al . [26] reported that sliding would dominate the bending for graphene nanoribbons, due to the low interlayer shear modulus. However, Koskinen [27] and Nikiforov et al . [35] found that when the edge of graphene nanoribbons was fixed, kinks and delamination became the major deformation mechanism. In our experiments, it was found that, while the free standing MoS 2 crystals are easy to slide, the interlayer sliding could be restricted by the interaction with the probes. The easy sliding could be understood by the low shear strength, which has been reported to be only around 0.1 GPa (refs 36 , 37 , 38 ). With a given maximum shear stress ( τ max ), the threshold bending angle for sliding can be calculated simply by applying the strength theory of materials [39] as , where L is the length, E is the Young’s modulus, N is the layer number and d is the interlayer distance. Therefore, the threshold angle is proportional to the square of length and inversely proportional to the square of layer number, as demonstrated in Supplementary Fig. 5 . For example, for an MoS 2 sheet with a length of 10 nm and five layers in thickness, the threshold angle would be as small as ~0.7°, which can explain the easy sliding during bending. It is also seen that when the length of the 2D crystal becomes larger it is more difficult to slide, which can explain why buckling rather than interlayer sliding became the major mechanism for bending the long BN and graphene nanoribbons with a length around 1 μm (ref. 35 ). Because of easy interlayer sliding, the atomic layers bend mostly independently, which is the reason for the minimum radius (corresponding to the maximum bending) to be non-related to the number of layers before the kinking mechanism comes into effect. The regarded 2D crystals might be bent to a radius as small as ~1.3 nm, showing that they are mechanically reliable candidates for future flexible electronic devices. For the 23-layer MoS 2 , we observed the appearance of kinking during bending, which is close to the deformation of the bulk crystals [28] , [29] . These kinks are different from the buckling and delamination phenomena discussed in the previous reports, where only the inner layers were buckled due to the compressive stress [27] , [35] . The formation of kinks could be understood by the competition between bending strain energy and commensurability effects in interfacial energy on interlayer sliding. The strain energy of a bent plate can be calculated using the following formula: , where M is the bending moment, I is the moment of inertia, b is the width, θ is the bending slope, N is the layer number and L is the length. When interlayer sliding occurs, the bending energy is N times that of one atomic layer and can be expressed as , which is proportional to N rather than to N 3 . Meanwhile, because of the interlayer sliding, the interfaces between the atomic layers become incommensurate and the increased interfacial energy can be calculated as , where γ int =0.11 N m −1 is the interfacial energy constant, L is the length of the sliding interface and c is the lattice constant along the sliding direction. It is reasonable to assume that the interfacial energy is a periodic function of the interlayer sliding distance [40] , [41] . 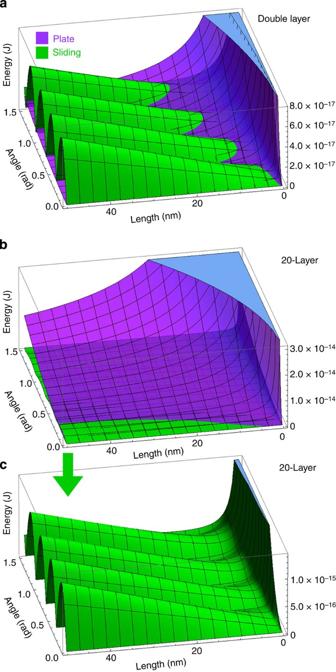Figure 5: Thickness-dependent energy competition during bending of 2D MoS2. (a,b) Calculated energy for double- and 20-layer MoS2. Bending strain energy corresponding to the plate-bending model is pictured purple. Combination of bending strain energy and interfacial energy for the bending-sliding model is pictured green. For the double-layer MoS2, the interfacial energy dominates and it tends to bend without interlayer sliding. For the 20-layer MoS2, the bending strain energy becomes dominating, and it tends to bend with interlayer sliding. (c) Detailed picture of the energy involved in the bending-sliding model for the 20-layer MoS2. Periodic nature of the interfacial energy with the bending angle is evident. Figure 5 demonstrates the calculated energy for double-, and 20-layer MoS 2 , where bending strain energy of the plate-bending model is pictured purple, and the combination of bending strain energy and interfacial energy related to the bending-sliding model is pictured green. For the double-layer MoS 2 , the interfacial energy dominates and it tends to bend without sliding ( Fig. 5a ). In constrast, for the 20 layer-MoS 2 , the bending strain energy becomes dominating, and it tends to bend with interlayer sliding ( Fig. 5b ). Figure 5c presents the detailed feature of the energy involved in the bending-sliding model for the 20-layer MoS 2 . Clearly, the interfacial energy is a periodic function of the bending slope. Therefore, for the thick MoS 2 flakes, during the sliding, when the interlayer sliding distance equals to the lattice constant or any other periodic distance along the sliding direction, the interfacial energy will show local minima. When the energy ‘valleys’ are met, abrupt force drop can be expected, which reflects the formation of kinks. It is noted that the period is around 0.36 rad (~20.6°), which is well consistent with our experimental observations. Figure 5: Thickness-dependent energy competition during bending of 2D MoS 2 . ( a , b ) Calculated energy for double- and 20-layer MoS 2 . Bending strain energy corresponding to the plate-bending model is pictured purple. Combination of bending strain energy and interfacial energy for the bending-sliding model is pictured green. For the double-layer MoS 2 , the interfacial energy dominates and it tends to bend without interlayer sliding. For the 20-layer MoS 2 , the bending strain energy becomes dominating, and it tends to bend with interlayer sliding. ( c ) Detailed picture of the energy involved in the bending-sliding model for the 20-layer MoS 2 . Periodic nature of the interfacial energy with the bending angle is evident. Full size image In conclusion, we developed an in situ TEM probing technique for direct investigation of the nanomechanical cleavage of 2D crystals. MoS 2 atomic layers were successfully cleaved from a single crystal with the layer number predetermined by the precise manipulation with an ultra-sharp probe. It was demonstrated that such cleavage is highly reversible. In addition, combining the in situ experiments with the MD simulations, the thickness-dependent mechanical behaviours were revealed. The featuring bending kinetics transformed from homogeneous curving and rippling (<5 atomic layers) to interlayer sliding (~10 layers) and to kinking (~20 or more atomic layers). Growth and characterization The MoS 2 atomic layers were synthesized on a SiO 2 /Si substrate by a vapour phase growth at 850 °C, using MoO 3 nanoribbons and pure sulphur as the precursors and reactants, respectively [21] . The crystalline structures of the MoS 2 atomic layers were characterized by TEM/STEM. The TEM samples were prepared by transferring the grown samples onto the TEM grids by direct contacting, so that the samples were free of contamination. The high-resolution TEM/STEM characterization was carried out on a FEI Titan [3] (Cube) microscope, equipped with a monochromator and Cs-correctors for probe-forming and imaging at an accelerating voltage of 300 kV in a HAADF imaging mode. In situ TEM probing experiments The in situ TEM probing experiments were mainly conducted using a scanning tunnelling microscope (STM)-TEM platform (‘Nanofactory Instruments AB’) in a HRTEM (JEM-3100FEF) with an accelerating voltage of 300 kV equipped with an OMEGA-type energy filter. Ultra-sharp tungsten probes (~10 nm tip diameter) were produced by electrochemical etching. MoS 2 single crystals were loaded on the edge of a gold wire with an edge-on orientation, and the tungsten tip movements were controlled by a piezoelectric motor to approach and selectively contact the atomic edge steps. After that, the tungsten tip was moved backwards to start the nanomechanical cleavage of the MoS 2 atomic layers. Bending deformation was then initiated by pushing the tungsten tip towards and along the edge of the MoS 2 crystal. The in situ force measurements were carried out by using AFM-TEM holder (‘Nanofactory Instruments AB’). The whole process was video recorded in real time by a charge-coupled device (CCD) camera. Simulation methods MD simulations were performed using the reactive empirical bond-order and Lennard-Jones potentials implemented into the Large-scale Atomic/Molecular Massively Parallel Simulator (LAMMPS) simulation package [42] . The Mo-S potential was parameterized to match density functional theory calculations of Mo, S and Mo-S structures [43] . The parameterization was successfully applied in the investigation of the mechanical properties of crystalline MoS 2 by the indentation method [44] and in the studies of behaviour of MoS 2 multilayered nanotubes in extreme pressure conditions [45] . This technique is perfect to describe structural and mechanical properties of the Mo-S systems consisting of a large number of atoms (>10 4 ). The MoS 2 systems were modelled as clusters with a length of ~40 nm (for mono- and 11- layer structures containing 1,400 and 13,300 atoms, respectively) and ~100 nm (for a 23-layer structure containing 19,500 atoms). In the case of mono- and 11-layer samples, the atoms on the end of the upper layers were fixed imitating the tip and moved along the direction corresponding to the experiment with a displacement step equal to 0.1 Å. In the case of 23-layer sample, for the imitation of the adhesion between the bottom edge of AFM tip and the sample, the MoS 2 monolayer of finite length was fixed and moved directly to the sample along the direction corresponding to the experiments with a displacement step equal to 0.1 Å. How to cite this article: Tang, D.-M. et al . Nanomechanical cleavage of molybdenum disulphide atomic layers. Nat. Commun. 5:3631 doi: 10.1038/ncomms4631 (2014).